Ultra-low carrier concentration and surface-dominant transport in antimony-doped Bi2Se3topological insulator nanoribbons A topological insulator is the state of quantum matter possessing gapless spin-locking surface states across the bulk band gap, which has created new opportunities from novel electronics to energy conversion. However, the large concentration of bulk residual carriers has been a major challenge for revealing the property of the topological surface state by electron transport measurements. Here we report the surface-state-dominant transport in antimony-doped, zinc oxide-encapsulated Bi 2 Se 3 nanoribbons with suppressed bulk electron concentration. In the nanoribbon with sub-10-nm thickness protected by a zinc oxide layer, we position the Fermi levels of the top and bottom surfaces near the Dirac point by electrostatic gating, achieving extremely low two-dimensional carrier concentration of 2×10 11 cm −2 . The zinc oxide-capped, antimony-doped Bi 2 Se 3 nanostructures provide an attractive materials platform to study fundamental physics in topological insulators, as well as future applications. The exotic electronic properties of the surface state, due to its spin-momentum-locked Dirac cone in the electronic band structure, define a topological insulator as a unique class of quantum matter [1] , [2] , [3] , [4] , [5] , [6] . Moreover, it is predicted to offer exciting physics, such as elusive quasi-particles, spin transport and fault-tolerant quantum information processing [1] , [2] , [3] , [4] , [5] , [6] , [7] , [8] , [9] . Bismuth selenide (Bi 2 Se 3 ) and its relative compounds are one of the most promising candidates to realize the ideal three-dimensional topological insulator due to their large bulk band gap and simple surface-band structure [10] . Significant advances have been made to probe the surface state in these materials by various methods, such as angle-resolved photoemission spectroscopy [11] , [12] , [13] and scanning-tunneling microscopy [14] , [15] , [16] . Transport measurements in bulk crystals have demonstrated the existence of these surface states as well [17] , [18] , [19] . Nanoscale topological insulator devices, with their large surface-to-volume ratio, offer a unique opportunity to manifest the surface effect [20] , [21] . In mesoscopic length scale, transport measurements may reflect the fundamental nature of carriers, as shown in previous cases like graphene [22] , [23] . However, it is still challenging to study the topological surface states in the device level, as material imperfections in the bulk blur transport signatures of the surface state and limit further in-depth studies. The major challenge is the dominance of bulk carriers outnumbering surface-state carriers, mainly originating from intrinsic Se vacancies [24] , [25] , [26] , [27] . Moreover, the material is very sensitive to environmental contamination—several studies observed that environmental exposure (H 2 O, O 2 ) causes material degradation and additional bulk carrier generation [17] , [28] . In this paper, we provide two effective solutions to eliminate both intrinsic and extrinsic sources of bulk carrier generation. First, we demonstrate vapour-phase antimony (Sb) doping in Bi 2 Se 3 nanoribbons systematically suppresses the bulk conductivity. Second, we show that a zinc oxide (ZnO) capping layer on Sb-doped nanoribbons can inhibit extra carrier generation induced by extrinsic contamination. Last, in an ultrathin device with Sb doping and ZnO capping, electrostatic manipulation allows us to locate the Fermi levels of both surfaces close to the Dirac point. The effective removal of bulk carriers achieves an ideal surface-transport state that is desirable for many applications of topological insulators. Vapour-phase Sb doping and bulk carrier suppression To suppress the bulk conductivity in topological insulator nanoribbons, we synthesize Bi 2 Se 3 nanoribbons with Sb doping. Sb is known as an effective compensation dopant to reduce bulk electron density to below 10 17 cm −3 in bulk crystals without destroying the topological surface state [17] , [29] . Bi 2 Se 3 nanoribbons are synthesized via vapour–liquid–solid growth mechanism using gold particles as catalysts [20] , [30] , and Sb vapour is introduced by the evaporation of an Antimony selenide (Sb 2 Se 3 ) powder placed at the lower temperature zone ( Fig. 1a ). As-grown ribbons are typically 50–300 nm thick, 200 nm to several micrometres wide, and up to tens of micrometres long ( Fig. 1b ). Sb-doped Bi 2 Se 3 nanoribbons are in a single crystalline rhombohedral phase ( Fig. 1c ), the same as undoped Bi 2 Se 3 nanoribbons. The distribution of Sb dopants is spatially uniform in the nanoribbon, as confirmed by energy-dispersive X-ray spectroscopy (EDX; Fig. 1c,d ). EDX spectra show simultaneous decreasing intensity of Bi peaks and increasing intensity of Sb peaks with higher Sb dopant concentrations ( Supplementary Fig. S1 ), suggesting the doping mechanism is likely the substitution of the Bi atoms by the Sb atoms. Assuming of the substitutional doping, we calculated the Sb doping level, ranging from 0 to 7%, in atomic ratio. 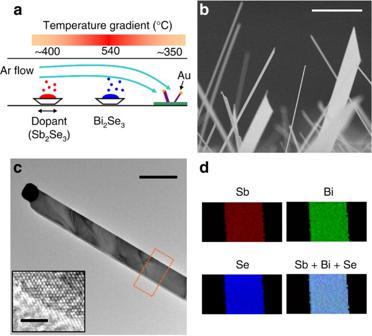Figure 1: Synthesis and material characterization of Sb-doped Bi2Se3nanoribbons. (a) A schematic of vapour–liquid–solid growth of Sb-doped Bi2Se3nanoribbons. By shifting the dopant source location along the temperature gradient in the tube furnace, the relative vapour pressures of two sources and the incorporated dopant level are controlled. (b) An scanning electron microscopy image of as-grown nanoribbons. Scale bar equals 10 μm. (c) A transmission electron microscopy image of a nanoribbon and its high-resolution image (inset). The rectangular box indicates the scanned area for EDX mapping. Scale bar equals 1 μm (Scale bar in the inset equals 2 nm). (d) Elemental maps of Sb (red), Bi (green), Se (blue) and overlaid RGB image by scanning EDX. The overlaid map looks bluish, as the Bi and Se signals are stronger than the Sb signal. The scanning map indicates homogeneous dopant distribution of 6% (atomic ratio) Sb with 0.5% s.d. Figure 1: Synthesis and material characterization of Sb-doped Bi 2 Se 3 nanoribbons. ( a ) A schematic of vapour–liquid–solid growth of Sb-doped Bi 2 Se 3 nanoribbons. By shifting the dopant source location along the temperature gradient in the tube furnace, the relative vapour pressures of two sources and the incorporated dopant level are controlled. ( b ) An scanning electron microscopy image of as-grown nanoribbons. Scale bar equals 10 μm. ( c ) A transmission electron microscopy image of a nanoribbon and its high-resolution image (inset). The rectangular box indicates the scanned area for EDX mapping. Scale bar equals 1 μm (Scale bar in the inset equals 2 nm). ( d ) Elemental maps of Sb (red), Bi (green), Se (blue) and overlaid RGB image by scanning EDX. The overlaid map looks bluish, as the Bi and Se signals are stronger than the Sb signal. The scanning map indicates homogeneous dopant distribution of 6% (atomic ratio) Sb with 0.5% s.d. Full size image The basic carrier types and densities of individual nanoribbons are measured by nanodevices with Hall bar geometry. Samples with different Sb concentrations ( Table 1 ) all show an n-type carrier-dominant transport, as their Hall resistances are negative values. By increasing the Sb dopant concentration, the sheet resistance increases more than an order of magnitude and the electron density is dramatically reduced, implying the significant decrease of bulk electron contribution ( Table 1 ). At a high Sb-doping concentration (6–7 atomic %), the carrier density is ~10 13 cm −2 . Considering the electron density of the surface states from the top and bottom surfaces near the bulk conduction band edge is ~10 13 cm −2 ( Supplementary Fig. S2 ), surface carriers are now expected to have the dominant role in transport of these Sb-doped nanoribbons. As a result, the two-dimensional (2D) carrier densities of nanoribbon devices are thickness-independent when the Sb doping is close to its maximum (6–7%; Supplementary Fig. S3 ). The surface-dominant transport is also supported by the comparable values of the averaged carrier mobility (Hall mobility) and field-effect mobility from the surface states in low-density samples ( Supplementary Table S1 ). Table 1 Full size table Additional electronic transport studies confirm that the bulk electron contribution is reduced significantly by the Sb doping. In Fig. 2a , temperature-dependent resistances from low Sb concentration samples (Sb 0–2%) follow typical metallic behaviour. In contrast, for the samples of high Sb concentration (Sb >4%), the resistance starts to increase and saturates at low temperature. An increase in resistance upon reducing temperature is likely due to the freeze-out of the bulk carriers. Moreover, electrostatic gating experiments in field-effect transistor devices manifest drastic difference between low and high Sb concentration samples ( Fig. 2b ). Low Sb-doped samples (Sb 0–2%) show weak gating dependence by a bottom gate, as the ribbon thicknesses (>70 nm) are much larger than the depletion layer thickness (~10 nm) with a relatively high carrier concentration. However, the gating response becomes larger with the increasing Sb-doping concentration. The sample with high Sb doping (T2, T3) exhibits large increase of its resistance and significant decrease in bulk carrier concentration. 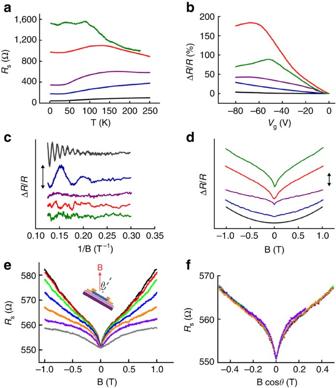Figure 2: Transport in nanoribbons without ZnO layer capping. (a–d) Transport measurement on nanoribbons of different doping concentration: undoped (B1, black), Sb 2% (B2, blue), Sb 4% (T1, purple), Sb 6% (T2, red), Sb 7% (T3, green). (a) The resistance profile versus temperature from Bi2Se3nanoribbons. We note that the curves for 4 and 7% Sb doping levels are from different devices of the same growth batch. (b) Gating response of the resistance from Bi2Se3nanoribbons (SiO2300-nm back gate). The resistance of high Sb concentration devices (purple, red, green) shows maximum peaks, indicating that the bottom surface switches from n-type to p-type. In general, devices of higher Sb concentrations reach the maximum peak at lower gating voltages, which suggests the Fermi level of the bottom surface to be closer to the Dirac point. (c) High-field MR versus inverse magnetic field (1/B). Background curve (either linear or parabolic) is subtracted from original MR curve. SdH oscillations from an undoped sample (BFFT~93 T) and 2% Sb sample (BFFT~22 T) correspond to bulk electron densities of ~6×1018and 6×1017cm−3, respectively. The arrow indicates 1% magnitude of total resistance. The curves are displayed with an offset for clarity. (d) MR near zero magnetic field, showing clear feature of weak anti-localization from samples of high Sb concentration (Sb >3%). The arrow indicates 2% magnitude of total resistance. Each curve is normalized by zero field resistance and displayed with an offset for clarity. (e) Angle-dependent MR (~5% Sb-doped sample,nH=2×1013cm−2,d=100 nm) with seven different field orientations: 0° (black), 15° (red), 30° (lime), 45° (blue), 60° (orange), 75° (purple), 90° (grey). Inset: a cartoon to describe the angle definition in the experiment. (f) MR with different field orientations, as a function of the perpendicular field component. All measurement are conducted at T=2 K except temperature-dependant studies. Figure 2: Transport in nanoribbons without ZnO layer capping. ( a – d ) Transport measurement on nanoribbons of different doping concentration: undoped (B1, black), Sb 2% (B2, blue), Sb 4% (T1, purple), Sb 6% (T2, red), Sb 7% (T3, green). ( a ) The resistance profile versus temperature from Bi 2 Se 3 nanoribbons. We note that the curves for 4 and 7% Sb doping levels are from different devices of the same growth batch. ( b ) Gating response of the resistance from Bi 2 Se 3 nanoribbons (SiO 2 300-nm back gate). The resistance of high Sb concentration devices (purple, red, green) shows maximum peaks, indicating that the bottom surface switches from n-type to p-type. In general, devices of higher Sb concentrations reach the maximum peak at lower gating voltages, which suggests the Fermi level of the bottom surface to be closer to the Dirac point. ( c ) High-field MR versus inverse magnetic field (1/B). Background curve (either linear or parabolic) is subtracted from original MR curve. SdH oscillations from an undoped sample ( B FFT ~93 T) and 2% Sb sample ( B FFT ~22 T) correspond to bulk electron densities of ~6×10 18 and 6×10 17 cm −3 , respectively. The arrow indicates 1% magnitude of total resistance. The curves are displayed with an offset for clarity. ( d ) MR near zero magnetic field, showing clear feature of weak anti-localization from samples of high Sb concentration (Sb >3%). The arrow indicates 2% magnitude of total resistance. Each curve is normalized by zero field resistance and displayed with an offset for clarity. ( e ) Angle-dependent MR (~5% Sb-doped sample, n H =2×10 13 cm −2 , d =100 nm) with seven different field orientations: 0° (black), 15° (red), 30° (lime), 45° (blue), 60° (orange), 75° (purple), 90° (grey). Inset: a cartoon to describe the angle definition in the experiment. ( f ) MR with different field orientations, as a function of the perpendicular field component. All measurement are conducted at T=2 K except temperature-dependant studies. Full size image The conductance of this ribbon decreases more than half by electrostatic manipulation via the bottom gate in spite of its large thickness (120 nm, T2), which strongly suggests the increase of the depletion layer depth (~35 nm) and the suppression of the bulk transport contribution. Its depletion-layer thickness can be estimated by two different ways, either by the Thomas–Fermi screening theory (for high carrier concentration) or solving the Poisson equation of charge-carrier density (for low carrier concentration). As the carrier density is low in most samples, we calculate the depletion layer thickness by solving band bending and do not consider the Thomas–Fermi screening theory. For undoped samples, the estimated depletion layer is ~10 nm, whereas for Sb-doped Bi 2 Se 3 nanoribbons of low carrier concentration, it is ~35 nm, according to the approximated expression . In the formula, κ is the dc dielectric constant of Bi 2 Se 3 (113), Δ E is the band-bending energy by gating, and n is the carrier density [24] , [31] . This number is based on the assumption that the carriers are distributed uniformly along the ribbon at zero gate voltage ( V g ). Magnetotransport data shows the emergence of the surface state and the suppression of bulk electrons by Sb doping. In the high-field magnetoresistance (MR), Shubnikov-de Haas (SdH) oscillations are observed in the samples of different Sb concentrations ( Fig. 2c ). The oscillations do not depend on the V g , which suggests that the oscillations originate from bulk electrons ( Supplementary Fig. S4 ). Without Sb doping, the small periodicity ( B FFT =93 T) of SdH oscillations in an inverse magnetic field corresponds to the large cross-sectional area of the bulk Fermi surface in a highly metallic sample with excessive bulk carriers. As the Sb concentration increases, the oscillation period gets larger ( B FFT =22 T) and disappears at high doping levels, because the bulk Fermi surface eventually becomes too small to be measured in our magnetic field range (8 T). The small cross section of the bulk Fermi surface corresponds to the decrease of the contribution of bulk electrons. It is reasonable to ask whether the heavy Sb doping dramatically degrades bulk electron mobility, so that the oscillation disappears. A previous study on bulk crystals showed strong bulk electron SdH oscillations observed from samples of heavy Sb doping, implying high electron mobility despite the large amount of dopants [17] . We also test the effect of doping on electron mobility, starting with a high Sb concentration sample (T3, without the ZnO layer initially) of low carrier concentration (10 13 cm −2 ). Within the 8 T range, we could not see any oscillatory features comparable to the SdH oscillations. Then, we put the ZnO layer (~10 nm) to protect the device from environmental doping during heating, and the sample was heat-treated at 100 °C for 4 h in moderate vacuum (~1 Torr argon gas-filled chamber). After the heat treatment, carrier concentration increased a lot (2.5×10 13 cm −2 ) and the SdH oscillations ( B FFT =17 T, E F =16 meV above the conduction band edge) emerged ( Supplementary Fig. S4 ). A temperature of 100 °C may not be regarded as a high-enough temperature to improve crystal quality, as we observed large carrier density increase from other samples, presumably by creating more Se vacancies. In this device, we also confirm that the Hall carrier density increases substantially. Therefore, we conclude that the electron mobility does not degrade by doping, and the fading of SdH oscillations is because of the elimination of bulk electrons. Weak anti-localization (WAL), the quantum correction in the spin-orbit-coupled surface state [25] , [32] , is absent in the MR trace of the undoped sample ( Fig. 2d , B1), as the large bulk electron contribution masks the surface-state transport. Samples with higher Sb concentration ( Fig. 2d , T1, T2, T3), in contrast, manifest the characteristic WAL as the sharp cusp near zero magnetic field due to the suppression of bulk conductivity. We conduct an angle-dependent study to verify the dominance of the 2D component in WAL; MR of a nanoribbon (Sb~5%) was measured at different field orientations ( Fig. 2e ). The cusp is the sharpest with the magnetic field perpendicular to the basal plane and becomes flatter as the angle ( θ ) increases. When the MR from different field orientations are plotted as a function of the perpendicular field ( B cos θ ; Fig. 2f ), they overlay nicely with the 0° MR, implying the observed WAL is essentially controlled by the 2D component. Additional fitting procedures are discussed in the Supplementary information ( Supplementary Fig. S5 , Supplementary Methods ). ZnO protective layer So far, we have shown that Sb doping effectively reduces bulk carriers. However, nanoribbons are still exposed to extrinsic contaminations during device fabrication, which can increase the bulk carrier concentration as well [17] , [28] . Therefore, we hypothesize that the intrinsic carrier density of the Sb-doped Bi 2 Se 3 should be much lower than that measured, and a protection layer is needed to access the intrinsic carrier density. We use ZnO for the protective layer due to the insulating properties of intrinsic ZnO, and its chemical stability against moisture and standard solvents in a wide range of temperature. Also, it can be deposited by a sputtering process without elevation of substrate temperature, avoiding additional Se vacancies generation upon heating. The sputtered ZnO layer covers the entire surface of the nanoribbons, which prevents degradation and extrinsic doping associated with the standard fabrication process. We compare carrier densities of 20 samples (10 with ZnO, 10 without ZnO capping) of different Sb concentrations ( Supplementary Fig. S6 ). On average, the ZnO-capped samples exhibit lower carrier densities than uncapped devices of similar Sb concentrations. Also, ZnO capping improves both the Hall mobility and the field-effect mobility. For samples of high Sb concentration (Sb=6–7%), the average Hall mobility of uncapped devices is ~500 (cm 2 V −1 s −1 ), whereas the average Hall mobility of ZnO-protected devices is ~750 (cm 2 V −1 s −1 ). In a bottom-gate device ( Fig. 3a ) fabricated on an Sb-doped, ZnO-protected nanoribbon of 200 nm in thickness, the carrier density is very low (~5×10 12 cm −2 ), and the gate-dependent resistance shows that the Fermi level of the bottom surface is close to the Dirac point even without applying the V g ( Table 2 ). In Fig. 3b , its resistance decreases by either direction of the gating voltage, and the Hall resistance increases due to the electrostatic accumulation of charge carriers at the bottom surface (p-type carriers for negative V g and n-type carriers for positive V g ). 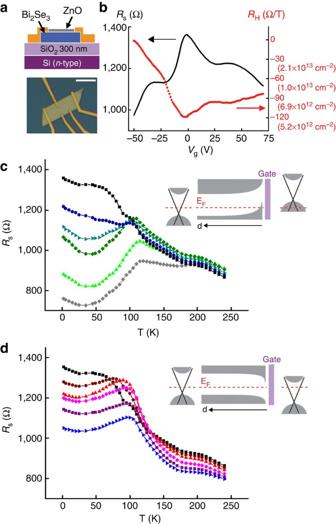Figure 3: Transport in a thick Sb-doped Bi2Se3nanoribbon with ZnO layer. (a) Device (Z1) schematic (top) and optical image (bottom) of a thick sample (200 nm) of Sb 7% concentration. Scale bar equals 5 μm. (b) Gate-voltage dependence of longitudinal sheet resistance (RS) and Hall resistance (RH) measured at low field (B<2 T) at T=2 K. Hall resistance increases in both direction ofVg, implying that the Fermi level of the bottom surface is near the Dirac point at zero gating voltage. The anomalous kink in the longitudinal resistance curve is not well understood, and it is not reproducible in other samples. (c) Temperature-dependent resistance curve at differentVg(negative): 0 V (black), −10 V (blue), −20 V (teal), −40 V (green), −60 V (lime), −80 V (grey). The curve changes significantly as more bulk holes are added, reflecting the conventional metallic temperature dependence of induced carriers. A band diagram (inset) shows band bending at the bottom surface induced by gating. (d) Temperature-dependent resistance curve at differentVg(positive): 0 V (black), +10 V (maroon), +20 V (red), +40 V (pink), +60 V (purple), +80 V (blue). In a band diagram (inset), the Fermi level does not cross any bulk band by positive gating, explaining the qualitatively similar temperature curves over the wide range of gating voltage. Figure 3: Transport in a thick Sb-doped Bi 2 Se 3 nanoribbon with ZnO layer. ( a ) Device (Z1) schematic (top) and optical image (bottom) of a thick sample (200 nm) of Sb 7% concentration. Scale bar equals 5 μm. ( b ) Gate-voltage dependence of longitudinal sheet resistance ( R S ) and Hall resistance ( R H ) measured at low field ( B <2 T) at T=2 K. Hall resistance increases in both direction of V g , implying that the Fermi level of the bottom surface is near the Dirac point at zero gating voltage. The anomalous kink in the longitudinal resistance curve is not well understood, and it is not reproducible in other samples. ( c ) Temperature-dependent resistance curve at different V g (negative): 0 V (black), −10 V (blue), −20 V (teal), −40 V (green), −60 V (lime), −80 V (grey). The curve changes significantly as more bulk holes are added, reflecting the conventional metallic temperature dependence of induced carriers. A band diagram (inset) shows band bending at the bottom surface induced by gating. ( d ) Temperature-dependent resistance curve at different V g (positive): 0 V (black), +10 V (maroon), +20 V (red), +40 V (pink), +60 V (purple), +80 V (blue). In a band diagram (inset), the Fermi level does not cross any bulk band by positive gating, explaining the qualitatively similar temperature curves over the wide range of gating voltage. Full size image Table 2 Transport parameters of Bi 2 Se 3 nanoribbon samples enclosed by ZnO layer (T=2 K, zero gate voltage) Full size table The gate-dependent temperature curve study also confirms that the Fermi level of the bottom surface is close to the Dirac point. The temperature-dependent resistance shows a non-metallic behaviour at zero V g , with the increase of resistance by lowering the temperature, and saturating at low temperature. By introducing holes with the negative V g ( Fig. 3c ), resistance starts to drop down by cooling (T<120 K), indicating the generation of bulk carriers, whereas the general behaviour does not change by inducing more electrons (positive V g , Fig. 3d ). The asymmetric temperature-dependent transport by different gating reflects the characteristic band structure near the Dirac point of Bi 2 Se 3 . From the angle-resolved photoemission spectroscopy studies [11] , [32] , the Dirac point of surface states is just above the bulk valence-band edge and far apart from the bulk conduction band edge (~0.2 eV). Within the range of V g (+80 V), positive gating only accumulates more electrons from the bottom surface band of the thick nanoribbon (inset of Fig. 3d ), which does not change the overall shape of the temperature curve. In contrast, bulk electronic states are easily populated from the valence band by negative gating (inset of Fig. 3c ), and the ribbon is in a mixed state with the coexistence of electrons and holes ( Supplementary Fig. S7 ). This temperature-dependent study confirms the independent tuning of the Fermi level of one surface near the Dirac point. Such a material system may allow the creation of a topological insulator junction of both types of carriers or a single surface junction to study novel proximity effects in the future [8] , [9] . Electrostatic manipulation of the Fermi level in an ultrathin device In addition to the manipulation of the bottom surface in the thick ribbons by substrate gating, the most attractive step is the flexible manipulation of the Fermi levels of both top and bottom surfaces, to position them close to the Dirac point. Such a control by electrostatic gating requires the nanoribbons to be thinned down. We etched a thick, Sb-doped ribbon (~100 nm) by argon plasma in a sputtering machine, and in situ deposited a 15-nm thick ZnO protection layer. In Fig. 4a , the ribbon is semitransparent with a thickness of 6 nm, more than 30 times thinner than the previous device ( Fig. 3 ). This device has a very low electron concentration of 2.8×10 12 cm −2 at zero V g ( Fig. 4b ), roughly four times lower than that (~10 13 cm −2 ) of the maximum density for pure surface conduction in the bulk band gap ( Table 2 ). Accordingly, the Fermi levels of both the top and bottom surfaces are completely within the bulk band gap. In other words, the Fermi level crosses only the surface Dirac cone above the Dirac point. 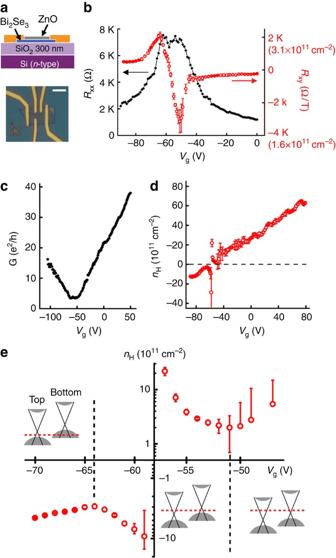Figure 4: Transport in an ultrathin Sb-doped Bi2Se3nanoribbon with ZnO layer. (a) Device (Z2) schematic (top) and optical image (bottom) of thin ribbon sample (6 nm) of Sb 5% concentration. Scale bar indicates 3 μm. (b)Vgdependence of longitudinal resistance (Rxx) and Hall resistance (Rxy) measured at low magnetic field (B<1 T), at T=2 K. Hall resistance decreases as n-type carriers are depleted (Vg>−50 V); increases as induced p-type carriers from the bottom surface form a mixed state with decreasing n-type carriers (−65 V<Vg<−50 V); and decreases again as the entire sample becomes a hole conductor (Vg<−65 V). (c) Conductance (G) versusVgcurve is linear, except near the minimum conductance (equivalent to the conductivity of 0.9 G0). (d) Electron density (nH) plot as a function ofVg. It depends onVglinearly in the wide range of voltage (−90 V to +80 V). (e) Semi-log scale plot of carrier density near its charge neutrality point (Dirac point). Band diagrams of top and bottom surfaces (inset) for samples with pure p-type conduction (left), mixed conduction (middle) and pure n-type conduction (right). Figure 4: Transport in an ultrathin Sb-doped Bi 2 Se 3 nanoribbon with ZnO layer. ( a ) Device (Z2) schematic (top) and optical image (bottom) of thin ribbon sample (6 nm) of Sb 5% concentration. Scale bar indicates 3 μm. ( b ) V g dependence of longitudinal resistance ( R xx ) and Hall resistance ( R xy ) measured at low magnetic field ( B <1 T), at T=2 K. Hall resistance decreases as n-type carriers are depleted ( V g >−50 V); increases as induced p-type carriers from the bottom surface form a mixed state with decreasing n-type carriers (−65 V< V g <−50 V); and decreases again as the entire sample becomes a hole conductor ( V g <−65 V). ( c ) Conductance (G) versus V g curve is linear, except near the minimum conductance (equivalent to the conductivity of 0.9 G 0 ). ( d ) Electron density ( n H ) plot as a function of V g . It depends on V g linearly in the wide range of voltage (−90 V to +80 V). ( e ) Semi-log scale plot of carrier density near its charge neutrality point (Dirac point). Band diagrams of top and bottom surfaces (inset) for samples with pure p-type conduction (left), mixed conduction (middle) and pure n-type conduction (right). Full size image In this ultrathin nanoribbon with very low carrier concentration, its small thickness of 6 nm makes it possible to shift the Fermi level of the entire ribbon by electrostatic gating across the Dirac point. By sweeping V g from positive to negative bias, its longitudinal resistance ( R xx ) initially increases and reaches a peak value (~7 kΩ) around V g of −50 V, and then decreases when further applying negative gate bias (black curve, Fig. 4b ). The corresponding Hall slope (red curve, Fig. 4b ) increases by more than ten times, and then switches the sign when R xx reaches the peak value. These results clearly demonstrate the ambipolar field effect and suggest that the entire sample is converted from n-type to p-type. The sample conductance depends on the gating voltage linearly, except at the plateau of minimum conductance (~3.6G 0 , equivalent to 2D conductivity of 0.9 G 0 , where G 0 is e 2 /h; Fig. 4c ). The absence of zero conductance region during the ambipolar transition is due to the gapless surface states. The carrier density obtained by the Hall resistance, shown in Fig. 4d , also linearly depends on V g . The sample remains purely n-type until V g =−50 V, switches to a mixed carrier state in the range of −65 V< V g <−50 V, and eventually to p-type when V g <−65 V ( Fig. 4e ). In the ultrathin device, the extremely low carrier density of n H =2×10 11 cm −2 observed at V g of −51 V indicates the Fermi levels of both surfaces simultaneously approach the Dirac point ( Supplementary Fig. S2 ). The removal of bulk electrons in topological insulator nanostructures achieves this stringent condition to study interesting physics near the Dirac point by transport. For example, the dimensional crossover by the top and bottom surface hybridization creates the surface band gap at the Dirac point and may possess exotic edge states [13] , [33] , [34] . Massive Dirac Fermions [35] and a new type of Hall effect [36] , by incorporation of magnetic dopants, will be another important physics near the Dirac point. Our experiment opens up the possibility that such interesting physics can be studied in nanoscale device transport, providing the material tunable near the Dirac point without excessive residual carriers. We also note that some studies propose that inhomogeneous Coulomb potential near the Dirac point [26] , [37] can contribute to the minimum carrier density, similar to the case of graphene [22] , [23] . It would be another interesting topic in topological insulator transport, and further study is expected to understand the observed minimum conductivity. Material synthesis and device fabrication The synthesis of Sb-doped Bi 2 Se 3 nanoribbons was carried out in a 12-inch horizontal tube furnace with a quartz tube. Bi 2 Se 3 source powder (99.999%) from Alfa Aesar was placed in the centre of the furnace; Sb 2 Se 3 source powder (99.999%) was placed at an upstream lower temperature zone; and the growth substrate, silicon wafer with thermally-evaporated 10 nm Au film, was placed at a downstream zone. High-purity argon gas was used to convey vapour from the source materials to a growth substrate at 130-s.c.c.m flow rate. During the entire growth time of 1.5 h, 1 Torr pressure and 540 °C centre zone temperature were maintained. The Sb dopant concentration in nano-ribbons can be controlled by varying the Sb 2 Se 3 source powder temperature—using the temperature gradient in the tube furnace; we placed the Sb 2 Se 3 source powder at different locations of the tube furnace, resulting in variation of the Sb 2 Se 3 source powder temperature. The estimated temperatures of the Sb 2 Se 3 source and the growth substrate are 450 and 350 °C, respectively, for the highest Sb concentration sample. After the vapour?liquid?solid growth, nanoribbons were directly transferred onto a doped silicon substrate with a 300-nm silicon dioxide layer. Then, a 15-nm thick ZnO layer was deposited by sputtering to cover the nanoribbon samples. In case of the thin ribbon sample, nanoribbons were etched by argon/metal plasma and capped by the ZnO layer in situ . The chemical composition and the surface roughness did not change with the Ar plasma etching, which were checked with Auger electron spectroscopy and atomic force microscopy (AFM). The nanoribbon devices were fabricated by standard e-beam lithography, and the ZnO layer on the contact area was etched by diluted base solution (tetra-methyl-ammonium hydroxide) followed by thermal evaporation of Cr/Au contact (5 nm/80 nm). The samples were stored in an N2 glovebox (H 2 O, O 2 <1 p.p.m.) at room temperature between processes. The device is usually measured within 1 or 2 days after device fabrication and 2 to 3 days after nanoribbon synthesis. Cryogenic transport measurement All transport measurements (except angle-dependant transport) were carried out in an Oxford 4 He cryostat with superconducting magnet, using low-frequency (~200–1 kHz) AC technique by digital lock-in amplifiers (Stanford Research Systems SR830) with current-driven configuration. Angle-dependant transport measurements were carried out in a Quantum Design PPMS-7 instrument, Janis 9T magnet He-cryostats (base temperature 2 K, low-frequency 1 kHz). A DC sourcemeter (Keithley 2400) was used to apply back V g with negligible leakage current (<1 nA). All samples were measured in either Hall-bar geometry or four-terminal configuration. The R xx curves were obtained by measuring the four-point resistance using the standard AC lock-in set-up while sweeping the V g continuously using the DC sourcemeter. Sheet resistances ( R s), conductivities and resistivities were obtained by measuring the device dimension by AFM/scanning electron microscopy. For the gate-dependent Hall measurement, we measured the Hall voltage at five different fields ( B =−1 T, −0.5 T, 0 T, 0.5 T, 1 T) while sweeping the gate and checked that the Hall slope is linear. The base temperature for all measurements was 2 K, except during the temperature-dependant studies. Material characterization For structural and elemental analysis, scanning transmission electron microscopy/transmission electron microscopy (FEI Tecnai G2 F20 X-Twin microscope, acceleration voltage 200 kV) equipped with an EDX spectrometer was used. The EDX spectra obtained from nanoribbons of different Sb concentrations are normalized to Se peaks (11.2 keV) for comparison. Typically, the EDX acquisition time was 300 s for all spectra for good signal-to-noise ratios ( Supplementary Fig. S1 ). Optical images were taken with Olympus BX51M and the scanning electron microscopy image was taken with FEI XL30 Sirion. AFM data were taken with Park Systems XE-70/XE-100. How to cite this article: Hong, S.S. et al . Ultra-low carrier concentration and surface-dominant transport in Sb-doped Bi 2 Se 3 topological insulator nanoribbons. Nat. Commun. 3:757 doi: 10.1038/ncomms1771 (2012).